Colossal resistance switching and band gap modulation in a perovskite nickelate by electron doping The electronic properties of correlated oxides are exceptionally sensitive to the orbital occupancy of electrons. Here we report an electron doping strategy via a chemical route, where interstitial dopants (for example, hydrogen) can be reversibly intercalated, realizing a sharp phase transition in a model correlated perovskite nickelate SmNiO 3 . The electron configuration of e g orbital of in SmNiO 3 is modified by injecting and anchoring an extra electron, forming a strongly correlated structure leading to the emergence of a new insulating phase. A reversible resistivity modulation greater than eight orders of magnitude is demonstrated at room temperature. A solid-state room temperature non-volatile proton-gated phase-change transistor is demonstrated based on this principle, which may inform new materials design for correlated oxide devices. Electron doping-driven phase transition accompanied by large conductance changes and band gap modulation opens up new directions to explore emerging electronic and photonic devices with correlated oxide systems. Correlated electron systems possess complex electronic phase diagrams that are exceptionally sensitive to the orbital occupancy of electrons and chemical/carrier doping. Particularly, electronic phase transitions observed in R NiO 3 perovskite nickelates (where R =rare earth lanthanide elements) are of broad interest in materials physics to understand band structure and oxide electronics such as but not limited to electronic switches [1] . The monotonic shift of carrier transport and magnetic properties with various 4f rare earth lanthanide elements correlated with the steric effect makes R NiO 3 an excellent platform in revealing the underlying correlated physics [2] . Conductance modulation in nickelates such as SmNiO 3 (SNO) as a result of the thermally driven insulator–metal transition is usually within one–two orders of magnitude right across the transition boundary [1] , [3] , [4] , which may originate from the subtle charge disproportionation (for simplicity, 2Ni 3+ →Ni (3+ δ )+ +Ni (3- δ )+ ) (refs 5 , 6 , 7 ). Spectroscopic characterizations reveal that the ground state of R NiO 3 has a strong covalency, described as in its insulating state [8] , [9] . Band gap opening accompanying such charge disproportionation, both theoretically and experimentally, scales to be at a few hundred millivolts [1] , [6] . Besides, the extremely short electrostatic screening length makes the resistance modulation challenging via electrostatic gating, as typical 10–30% carrier doping per unit cell is required to induce a phase transition even with ionic liquids [10] , [11] , [12] , [13] , [14] . Herein, we demonstrate an electron doping-driven phase transition of SNO via a chemical route. By manipulating the electron configuration of e g orbital of SNO, we have discovered a reversible colossal resistance switching and optical band gap modulation in the correlated oxide SNO. The phase transition accompanies a resistivity modulation of more than eight orders of magnitude and an order of magnitude change in optical band gap at room temperature. The modulation mechanism is verified and manifested by three different electron doping systems. A solid-state room temperature proton-gated phase-change transistor has been demonstrated utilizing the reversible and non-volatile switching behaviour, which can open new directions in exploring correlated oxide devices. Proposed phase transition mechanism During the thermally driven phase transition in SNO, the NiO 6 octahedron buckles at below metal–insulator transition (MIT) temperature, which reduces the orbital overlapping and renders an insulating phase ( Fig. 1a ) [15] . Charge disproportionation is mostly proposed as the cause for SNO’s insulating phase ( Fig. 1b ) [6] . The formulated expression of charge disproportionation can be simplified for convenient description as , which neglects the covalent character of the ground state but can qualitatively reflect the physical process [6] . Integer valence values are used here to represent the quantum numbers of the respective states rather than the actual charges [6] . 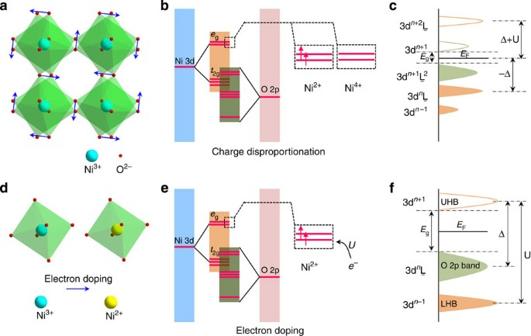Figure 1: Principle of charge disproportionation and electron doping-driven colossal phase transition in SmNiO3(SNO). (a) Buckling of NiO6octahedra in SNO is a structural manifestation along with the MIT. (b) Molecular orbitals of SNO insulator with charge disproportionation. (c) A schematic band diagram of SNO in its insulating state proposed as negative charge-transfer insulator with Ni ions with charge disproportionation configuration.Egis the band gap andUis the d–d Coulomb and exchange interactions. (d) Electron doping-induced reduction of Ni3+to Ni2+. (e) Molecular orbitals of electron-doped SNO in its insulating phase with Ni2+replacing Ni3+. (f) Band diagram shows the charge-transfer electron-doped SNO insulator with Ni2+inconfiguration.Egis the band gap andUis the d–d Coulomb and exchange interactions. Figure 1b shows the corresponding electron configuration of the charge-ordered Ni 2+ and Ni 4+ sites with crystal field-induced e g orbital in the insulating phase. The doubling of unit cell and combination of and render a new band diagram with a Mott–Hubbard splitting involved. Though there is a debate about whether nickelates are Mott–Hubbard insulator [16] , charge-transfer insulator [17] , negative charge-transfer insulator [18] or even band insulator [6] , both theoretical and experimental evidence indicate such band gap of SNO’s insulating state is quite small (a few hundred millivolts) because of the mixed character of Ni 2+ and Ni 4+ (or Ni (3- δ )+ and Ni (3+ δ )+ ). As an example, Fig. 1c shows the band diagram of nickelates simplified as a negative charge-transfer insulator, whose band gap is manifested by the electron transfer within oxygen p–p bands. Nevertheless, in either case of these proposed insulator types, the small band gap of SNO fundamentally limits the magnitude of the conductance modulation by thermal-driven phase transition. Figure 1: Principle of charge disproportionation and electron doping-driven colossal phase transition in SmNiO 3 (SNO). ( a ) Buckling of NiO 6 octahedra in SNO is a structural manifestation along with the MIT. ( b ) Molecular orbitals of SNO insulator with charge disproportionation. ( c ) A schematic band diagram of SNO in its insulating state proposed as negative charge-transfer insulator with Ni ions with charge disproportionation configuration. E g is the band gap and U is the d–d Coulomb and exchange interactions. ( d ) Electron doping-induced reduction of Ni 3+ to Ni 2+ . ( e ) Molecular orbitals of electron-doped SNO in its insulating phase with Ni 2+ replacing Ni 3+ . ( f ) Band diagram shows the charge-transfer electron-doped SNO insulator with Ni 2+ in configuration. E g is the band gap and U is the d–d Coulomb and exchange interactions. Full size image Rather than forming a charge disproportionation, we herein propose an electron doping strategy by chemical route to inject an extra electron to the e g orbital of Ni 3+ of SNO’s metallic phase to drive a phase transition. With one more electron, converts to of high spin configuration in e g orbitals due to Coulomb repulsion under the octahedron framework ( Fig. 1d,e ) [19] . The strong Coulomb repulsion (d–d Coulomb and exchange interactions is defined as U) between electrons in the single e g orbital of (when one electron is lost or gained due to the process: 3d n +3d n →3d n −1 +3 n +1 ) induces a large Mott–Hubbard splitting ( Fig. 1f ). This is in sharp contrast to the case of Ni 3+ where charge disproportionation in Ni 3+ does not create doubly occupied state and therefore only induces a very small band gap. Consequently, such splitting helps to create a much larger band gap, typically several electron-volts even in charge-transfer insulators [20] . Due to the exponential decay in the number of thermal-activated carriers with respect to the magnitude of insulating band gap, a much larger conductance modulation can be achieved by electron doping strategy. To enable electron doping on Ni ions, reducing chemical species such as hydrogen or metals of small ionic radii with lower electronegativity than Ni are utilized, by which a proton or small metal cation often binds with oxygen anion and electron goes to the orbital of heavy metal ion of parent materials. This often occurs in electrochromic binary oxides, such as WO 3 (ref. 21 ). Electron doping-induced phase transition by hydrogenation Single-crystal lanthanum aluminate (LAO) or Si with a thermal oxide (300 nm thick) were used as the growth substrate. A combination of sputtering and ultrahigh pressure annealing was utilized for sample preparation (as the phase is not stable in ambient conditions) [3] . We synthesize samples by co-sputtering from metallic Sm and Ni targets in Ar/O 2 atmosphere, which allows us to precisely control the cation ratio. Complete experimental details can be found in Methods. The SNO/LAO or SNO/SiO 2 /Si samples were then patterned with Pt electrode arrays with the width of each bar 250 μm and their intervals 500 μm, as shown in Fig. 2a . The Pt serves as a catalyst, which dissociates hydrogen during hydrogenation process. 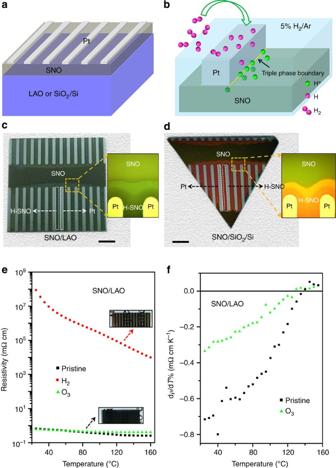Figure 2: Hydrogenation of SNO. (a) A schematic illustration of Pt catalyst patterned on SNO film grown on LAO or SiO2/Si substrate, where the space between adjacent Pt bars is 600 μm in width. (b) Proton intercalation process catalysed by Pt via the triple phase boundary. (c) A photo of hydrogenated SNO on LAO. On the region (marked as ‘SNO’) further away from Pt bars, the sample displays a dark grey colour, which is identical to the pristine one. In the space between Pt bars (marked as ‘H-SNO’), the sample becomes translucent. Scale bar, 2 mm. Right inset shows the optical image of the transient region. (d) A photo of hydrogenated SNO on SiO2/Si. In the vicinity of Pt bars, the sample colour changes to red, while the sample further away from Pt retains its original colour. Scale bar, 2 mm. Right inset shows the optical image of the transient region. (e) Resistivity versus temperature of pristine, hydrogenated and ozone-annealed SNO on LAO sample, respectively, recorded in air. Insets are the corresponding photo images (marked by the respective arrows). (f) Derivative of resistivity versus temperature plotted as a function of temperature of pristine and ozone-annealed SNO on LAO sample recorded in air. Figure 2b schematically illustrates the proposed proton intercalation process in SNO. At the triple phase boundary (Pt-SNO-H 2 /Ar), H 2 first dissociates to atomic hydrogen and then splits to H + and e − , which are incorporated into SNO lattice. The samples were loaded in a home-made annealing chamber and heated at 200 °C in hydrogen atmosphere (5% H 2 in Ar). On hydrogen annealing, for the SNO/LAO sample, SNO regions in the vicinity of Pt bars become optically translucent (indexed as H-SNO in Fig. 2c ), while the region further away from the Pt bars is still in its original dark colour (indexed as SNO). In Fig. 2d , we present the hydrogenation effect on the SNO/SiO 2 /Si sample. SNO regions near Pt bars appear red and further away still retain the original dark colour. Optical microscope was used to image the details of the H-SNO, SNO and the transition regions (insets of Fig. 2c,d ). Distinct colour contrast was spotted between H-SNO and SNO regions. The gradual colour change from SNO to H-SNO region is due to the diffusional proton transport in SNO. Figure 2: Hydrogenation of SNO. ( a ) A schematic illustration of Pt catalyst patterned on SNO film grown on LAO or SiO 2 /Si substrate, where the space between adjacent Pt bars is 600 μm in width. ( b ) Proton intercalation process catalysed by Pt via the triple phase boundary. ( c ) A photo of hydrogenated SNO on LAO. On the region (marked as ‘SNO’) further away from Pt bars, the sample displays a dark grey colour, which is identical to the pristine one. In the space between Pt bars (marked as ‘H-SNO’), the sample becomes translucent. Scale bar, 2 mm. Right inset shows the optical image of the transient region. ( d ) A photo of hydrogenated SNO on SiO 2 /Si. In the vicinity of Pt bars, the sample colour changes to red, while the sample further away from Pt retains its original colour. Scale bar, 2 mm. Right inset shows the optical image of the transient region. ( e ) Resistivity versus temperature of pristine, hydrogenated and ozone-annealed SNO on LAO sample, respectively, recorded in air. Insets are the corresponding photo images (marked by the respective arrows). ( f ) Derivative of resistivity versus temperature plotted as a function of temperature of pristine and ozone-annealed SNO on LAO sample recorded in air. Full size image Figure 2e presents the colossal resistance change of SNO on its exposure to hydrogen. All the resistivity–temperature ( R – T ) data were collected in ambient atmosphere. Pristine SNO on LAO shows a typical MIT characteristic (see Supplementary Fig. 1 ) with its transition temperature at ~140 °C, close to its bulk value [2] . The resistivity of pristine SNO at 25 °C is 0.6 mΩ cm. On 15 min 5% H 2 /Ar annealing at 200 °C, the resistivity of SNO sample (at room temperature) increases to 10 8 mΩ cm and is quite stable at ambient conditions. As shown in inset of Fig. 2e , we barely see the words underneath the pristine SNO/LAO sample (bottom), while the words are clearly visible under the annealed sample (top) in the region catalysed by Pt strips (the darker lines). The resistivity retention of SNO sample annealed (in H 2 /Ar) at 100 °C was recorded as well (see Supplementary Fig. 2 ). Such hydrogenation process yields a colossal resistance change of >10 8 and non-volatility. The resistivity of H-SNO drops as the temperature increases, indicating an insulator-like behaviour. It should be noted that its resistivity drop is attributed to the hydrogen extraction in air (that is, opposite to hydrogen intercalation) at high temperatures. Nevertheless, after ~6 h of temperature cycling between 25 °C and 165 °C in air, the resistivity of H-SNO is still above 10 5 mΩ cm. To fully recover the resistivity, we anneal the H-SNO sample in O 3 (a highly oxidizing environment) for 10 h at 300 °C. Varied annealing temperatures and durations were attempted to explore the resistivity recovery properties (see Supplementary Fig. 3 ). R – T measurement shows that its resistivity returns to the normal value for stoichiometric SNO. It should be noticed that samples annealed in air at 200 °C for a long period of time could recover to the normal SNO state as well (see Supplementary Fig. 3 ). For the nickelates in general, the MIT temperature is defined by the sign change in temperature coefficient of resistivity, from d ρ /d T <0 (insulating state) to d ρ /d T >0 (metallic phase). d ρ /d T versus T shown in Fig. 2f exhibiting a MIT temperature 130~140 °C (defined by the change of sign) confirms the recovery of SNO to its initial state. Cycling testing by following above annealing path gives us reproducible results. Identical measurements were also conducted on SNO/SiO 2 /Si and SNO/GeO x /Ge samples, showing similar performance. R – T plots for both pristine and hydrogenated SNO samples over an extended temperature widow are shown in Supplementary Fig. 4 . It should be noted that without Pt electrodes, there is no significant change in the resistivity or R – T characteristic of SNO after hydrogen annealing under identical conditions (see Supplementary Fig. 5 ). Real-time measurements were conducted to monitor the resistivity evolution during the hydrogen annealing process ( Fig. 3a,b ). Before the measurement, the sample (SNO/SiO 2 /Si) was sealed in a pure Ar filled chamber. The resistivity is monitored versus time immediately after the H 2 /Ar gas is introduced into the chamber at 150 sccm flow rate. Initially at 20 °C, the resistivity of the sample increases drastically from 10 0 mΩ cm to 10 3 mΩ cm within 10 min ( Fig. 3a ). The resistivity then slowly increases for ~10 min, after which it shoots up quickly again and reaches a constant value (>10 6 mΩ cm), rendering a final on/off ratio of more than six orders of magnitude. By turning off H 2 and introducing O 2 and O 3 in sequence at 20 °C, the resistivity recovers to its original value. At 50 °C, a similar phenomenon was observed after the introduction of H 2 /Ar except that the whole transition process proceeds faster than at 20 °C ( Fig. 3b ). When its resistivity reaches a high value (>10 6 mΩ cm), H 2 was turned off and Ar was introduced to unveil SNO’s non-volatility in inert atmosphere. The resistivity stabilizes (>10 4 mΩ cm) in an asymptotical manner. Immediately after the purge of O 3 , the resistivity returns to its original value after a few hours similar to the 20 °C case. The extreme sensitivity of SNO to proton intercalation at various temperatures (ranging from room temperature to at least 200 °C) makes it a rather interesting candidate for hydrogen sensing, ionically mediated switching and synaptic electronics compatible with CMOS technologies. It should be noticed that, along the resistivity ramp path both at 20 and 50 °C, there is always a short ‘stand’ where resistivity escalates quite slowly. This ‘stand’ region begins at 5 × 10 2 mΩ cm at 20 °C and 1 × 10 2 mΩ cm at 50 °C. The emergence of this region suggests the possible existence of a metastable H-SNO phase with varying hydrogen concentration in SNO. 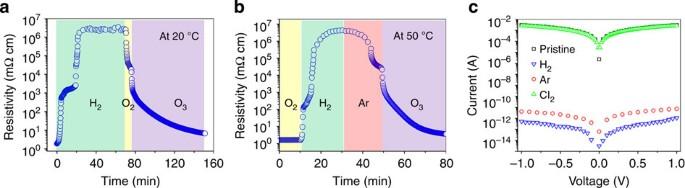Figure 3: Resistivity evolution under different annealing conditions. (a) Resistivity of SNO versus time exposed in H2, O2and O3in sequence at 20 °C. (b) Resistivity of SNO versus time exposed in O2, H2, Ar and O3in sequence at 50 °C. (c)I–Vcharacteristics of pristine SNO and samples annealed in H2, Ar and Cl2. Figure 3: Resistivity evolution under different annealing conditions. ( a ) Resistivity of SNO versus time exposed in H 2 , O 2 and O 3 in sequence at 20 °C. ( b ) Resistivity of SNO versus time exposed in O 2 , H 2 , Ar and O 3 in sequence at 50 °C. ( c ) I – V characteristics of pristine SNO and samples annealed in H 2 , Ar and Cl 2 . Full size image To confirm that the drastic change of electrical conductivity arises from proton intercalation rather than oxygen vacancy formation, control experiments have been conducted as shown in Fig. 3c . After the hydrogenated sample (the hydrogenation was conducted at 200 °C for 30 min) was annealed in chlorine gas at 200 °C for 5 min, its electrical conductivity recovered to that of a pristine sample (displaying the characteristic thermal-induced insulator–metal transition). This is consistent with what is observed when the hydrogenated sample was annealed in O 2 and O 3 . To rule out the impact of trace oxygen during Cl 2 annealing process, the hydrogenated sample was also annealed in pure Ar under identical conditions. As shown in Fig. 3c , the hydrogenated sample annealed in Ar showed only a very slight change in resistivity. To reveal the crystal structure evolution on hydrogenation, samples for cross-sectional transmission electron microscopy (XTEM) were specially prepared by focused ion beam (FIB) milling followed by proton intercalation. Pt was deposited in the vicinity of SNO region of the TEM sample to enable effective proton intercalation during hydrogen annealing (see Supplementary Fig. 6 ). Electron diffraction patterns show that the crystal structures of pristine SNO ( Fig. 4a ) and H-SNO prepared by hydrogenation at 200 °C for 15 min ( Fig. 4b ) are identical within the resolution of the technique. After O 3 annealing at 300 °C for 10 h to recover SNO’s resistivity, its crystal structure remains unchanged as well ( Fig. 4c ). High-resolution X-ray diffraction (XRD) was performed to confirm the epitaxial relationships between SNO film and LAO substrate and the polycrystalline nature of SNO on SiO 2 /Si substrate (see Supplementary Fig. 7 ). High-resolution XRD characterization also indicated no noticeable change of lattice parameters of SNO on hydrogenation (see Supplementary Fig. 7 ). Phi-scans were also conducted to confirm the epitaxy, manifested by four equally spaced (202) orthorhombic reflections from the film as shown in Fig. 4d (SNO film and LAO substrate are indexed with orthorhombic and pseudocubic notations, respectively.). The epitaxial relationship determined by XRD is consistent with that obtained by electron diffraction. Hence, there is no drastic structural transition accompanying this resistance change. Atomic force microscopy experiments on the various samples indicate similar surface morphology (see Supplementary Fig. 8 ). The mechanism of proton intercalation and conductivity modulation is therefore independent of the single versus polycrystalline nature of the film. X-ray photoelectron spectroscopy (XPS) characterization on pristine and hydrogenated samples reveals that the major Ni(2p3/2) peak shifts to lower binding energy state after intercalation (no noticeable change observed on Sm 3+ peaks), suggesting qualitatively a relative increase of Ni 2+ fraction and decrease of Ni 3+ in H-SNO ( Fig. 4e ) [22] . Further analysis and comparison with literature is presented in Supplementary Fig. 9 and Supplementary Table 1 . The complex refractive indices of pristine and hydrogenated SNO were obtained by variable-angle Ellipsometry ( Fig. 4f and see Supplementary Fig. 10 ). The dielectric function of LAO substrate was acquired on a bare 1-mm thick LAO substrate and modelled with a commonly used Cauchy dispersion relation for transparent materials. The thickness of SNO film (80 nm) measured by cross-sectional TEM was used in the data fitting to reduce the unknown parameters and over-fitting errors. The dispersion of both SNO and H-SNO were modelled by a general classical oscillator model with contributions from high-frequency dielectric constant, free electron oscillation and resonant absorption due to lattice vibrations and interband transitions. The fitted dielectric function of pristine SNO shows character of free electron absorption and dipolar absorption at low and high frequencies respectively [23] . Using the Drude model to fit the long wavelength tail, resistivity of pristine SNO was estimated to be ~0.7 mΩ cm, in good agreement with electrical measurements (~1 mΩ cm). The higher energy characters could be related to band to band transition in SNO. On the other hand, the optical constants of H-SNO from 3 to 5 eV are characterized by a typical oscillator function of absorbing materials. The sharp increase in the absorption indicates an optical band gap of approximately 3 eV for H-SNO. Below 3 eV, the absorption is close to but not exactly zero due to residual SmNi [3+] O 3 phase in the matrix. 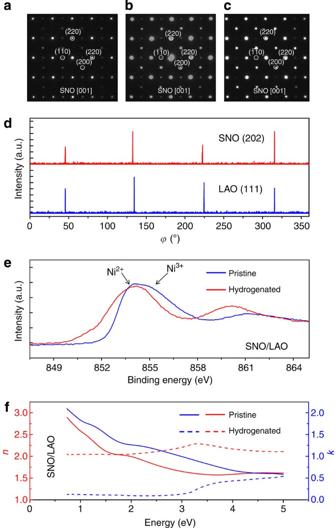Figure 4: Structural analysis and possible mechanism of proton-driven MIT. Electron diffraction patterns of (a) pristine, (b) proton-intercalated, (c) ozone-annealed SNO sample. (d) XRDφ-scan of SNO grown on LAO (SNO and LAO are indexed in orthorhombic and pseudocubic, respectively). (e) X-ray photoelectron spectra of pristine and hydrogenated samples qualitatively indicating an increase in Ni2+fraction after hydrogen annealing of SNO at 200 °C for 15 min. (f) Complex refractive indices of pristine and hydrogenated SNO from variable-angle ellipsometry. Figure 4: Structural analysis and possible mechanism of proton-driven MIT. Electron diffraction patterns of ( a ) pristine, ( b ) proton-intercalated, ( c ) ozone-annealed SNO sample. ( d ) XRD φ -scan of SNO grown on LAO (SNO and LAO are indexed in orthorhombic and pseudocubic, respectively). ( e ) X-ray photoelectron spectra of pristine and hydrogenated samples qualitatively indicating an increase in Ni 2+ fraction after hydrogen annealing of SNO at 200 °C for 15 min. ( f ) Complex refractive indices of pristine and hydrogenated SNO from variable-angle ellipsometry. Full size image The colossal resistance modulation, XPS, band gap opening and switching of complex refractive index unanimously indicate that there is a phase transition involving the shift of the valence charge or Ni–O bonding character on hydrogenation while the parent framework remains unchanged. These observations agree well with the expectation when in SNO converts to . During the hydrogenation process, on the triple phase boundary, protons dissociated from hydrogen molecules diffuse to SNO and specifically often go to the neighbourhood of oxygen ions and electrons from hydrogen due to charge neutrality join the e g orbital of Ni 3+ forming a Ni 2+ electron configuration. The phase transition occurring at 20 and 50 °C demonstrated herein indicates such electron configuration shift is thermodynamically preferable when a large quantity of electron donor is provided. This is reasonable from synthesis perspective and consistent with SNO’s phase diagram. Conventionally, to establish Ni 3+ dominant phase in SNO, either extreme high O 2 pressure (above 100 bars) at intermediate temperature or epitaxial strain (induced by the lattice mismatch between substrates and SNO) is necessary [3] , [4] . The thermodynamic properties of Ni 3+ and Ni 2+ makes it feasible to induce phase transitions through electron doping near room temperature. Doping-induced phase transition by Li and Mg intercalation Aside from hydrogen, electron donor alkaline metal Li was investigated to verify our hypothesis. Electrons from the metal can be incorporated into the e g orbital of Ni 3+ to form a Ni 2+ of high spin configuration in the e g orbital and Li + binds with oxygen ion. Such a process is expected to be able to reproduce the observations in hydrogenated SNO. 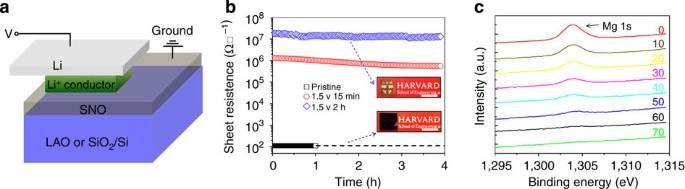Figure 5: Electron doping-driven phase transition in SNO via Li intercalation. (a) A schematic showing Li intercalation in SNO. (b) Resistance change and visual appearance modification of Li-intercalated SNO at different times. The non-volatile property is indicated by the plots of sheet resistance versus time. Scale bar, 1 cm. (c) Depth-dependent X-ray photoelectron spectra of Mg-intercalated SNO film grown on LAO substrate. The experimental conditions for intercalation are identical to that ofSupplementary Fig. 12. Inset legends indicate the depth into the film (unit: nm). Figure 5a is the schematic drawing of the electron doping of SNO via Li intercalation utilizing an electric double layer transistor device (or an electrochemical cell). With a Li + electrolyte (saturated lithium perchlorate in propylene carbonate) shuttling Li + between a Li metal plate gate and SNO, Li intercalation of SNO could proceed when a large enough positive bias is applied to the Li metal. Figure 5b graphs the change of the sheet resistance of SNO on Li intercalation. The pristine SNO shows a sheet resistance of 120 Ω per square and it increases to above 10 6 Ω per square with 15 min gating at 1.5 V. When the gating duration reaches 2 h at 1.5 V bias, the sheet resistance is above 10 7 Ω per square. Drastic optical transition (from dark of pristine sample to translucent of 2 h gating sample) is also noted along with the resistance switching (inset of Fig. 5b ). Both the electrical and optical phase transitions of SNO with Li intercalation are very similar to what is seen in our hydrogenation experiments, which supports our proposed model. The reversibility and non-volatility of the SNO phase transition triggered by Li intercalation/deintercalation is shown in Supplementary Fig. 11 . The above results indicate that the colossal phase transition is indeed driven by electron doping and could be universal with other electron dopants when the parent SNO crystal structure is maintained. In addition, different doping concentration and spatial distribution can also lead to different transport properties, because different phases can emerge in different doping regimes in complex oxides. To further verify this hypothesis, Mg intercalation experiments were carried out in a similar manner (see Supplementary Fig. 12 ). This further allowed the quantification of doping concentration as the lighter elements, namely H and Li are challenging to analyse by energy-dispersive spectroscopy and XPS. Depth-dependent XPS spectra taken from SNO thin films intercalated with Mg under identical conditions as in Supplementary Fig. 12 indicate their presence well into 50 nm depth from the surface ( Fig. 5c ). This further supports the phase transition being mediated by electron doping from donor elements such as H, Li and Mg into SNO rather than oxygen vacancy formation. In addition, to verify that it is Li or Mg intercalated into SNO, secondary ion mass spectrometry (SIMS) experiments were conducted to reveal the distribution of Li, Mg, O, Sm and Ni along the thickness of the film (see Supplementary Fig. 13 ). It is seen that the oxygen composition remains constant across the depth direction within the measurement limits, while Li and Mg exhibit a depth-dependent distribution. It has been found previously the insulating phase of NdNiO 3 (NNO) can be suppressed by substitutional dopants such as Ce and Th at low-doping concentration [24] . However, it should be noted that cationic steric effects also play a role for modulating transport properties in NNO, while it is primarily an electronic effect in the present study. To demonstrate the difference of these two types of dopants (Ce and H herein) in SNO film, we conducted Ce doping on our SNO film and then annealed the Ce-doped SNO film in hydrogen. As shown in Supplementary Fig. 14 , Ce-doped SNO exhibits suppressed phase transition temperature consistent with previous studies [24] . After Ce-doped SNO is annealed in hydrogen, greater than seven orders change in resistivity is observed, which is consistent with our observation on pristine SNO. The atomic ratio of cation doping (in ref. 24 ) to Ni is maximum at 0.10, while the local doping concentration approaches nearly one H/Li (or 0.5 Mg) per Ni in the vicinity of the film surface (derived based on energy-dispersive spectroscopy/XPS data and SIMS profile). Figure 5: Electron doping-driven phase transition in SNO via Li intercalation. ( a ) A schematic showing Li intercalation in SNO. ( b ) Resistance change and visual appearance modification of Li-intercalated SNO at different times. The non-volatile property is indicated by the plots of sheet resistance versus time. Scale bar, 1 cm. ( c ) Depth-dependent X-ray photoelectron spectra of Mg-intercalated SNO film grown on LAO substrate. The experimental conditions for intercalation are identical to that of Supplementary Fig. 12 . Inset legends indicate the depth into the film (unit: nm). Full size image Solid-state protonic SNO transistor To verify that it is the proton and not negative hydrogen ion (such as observed in YH 3- δ ) [25] or oxygen vacancies [26] , which diffuses in SNO and also to demonstrate a proof-of-concept solid-state field effect device, a proton-gated transistor is fabricated, as shown in Fig. 6a . We start with a pristine SNO bar patterned on LAO by photolithography. Two Pt electrodes are sputtered on SNO as the source and drain terminal. Pt also serves as catalyst for hydrogen dissociation. Then a low-temperature proton conductor yttrium-doped barium zirconate (BYZ) is grown on top that serves as a proton reservoir/conductor to store/transport protons [27] . Above it, yttria-stabilized zirconia (YSZ) is deposited to serve as a gate insulator at device operation temperature. The low proton conductivity in YSZ at room temperature makes it a good barrier to prevent protons leaving from BYZ/SNO gate stacks during device operation at 20 °C; its relatively high proton conductivity at elevated temperature makes it possible to inject protons through the Pd gate electrode into BYZ/SNO layers at elevated temperature [28] . On YSZ, Pd gate electrode serves as both excellent proton conductor and catalyst for hydrogen dissociation [29] . Detailed fabrication process can be found in Methods. The working principle of such proton transistor is illustrated in Fig. 6b . First, hydrogen molecules dissociate at the gate electrode and the protons diffuse into BYZ and SNO, as illustrated in the left inset of Fig. 6b . The proton diffusion process proceeds preferably at elevated temperature, for example, at 200 °C, due to enhanced ionic conductivity of BYZ and YSZ. Below 100 °C, during hydrogenation process, due to the existence of a proton conduction barrier YSZ, SNO’s resistivity is barely modulated. At 200 °C, SNO resistivity increases by several orders in less than one minute. Second, when a negative bias is applied to the Pd gate electrode, the majority of protons in SNO are attracted to BYZ under the electric field, as illustrated in the middle inset of Fig. 6b . At this state, the SNO body protons are removed and Ni 3+ recovers due to charge neutrality. Its resistivity is low and the transistor’s state is ‘on’. When a positive bias is applied, protons are pushed to SNO body, which is accompanied by the reduction of Ni 3+ to Ni 2+ resulting in a high resistivity state of SNO, that is, transistor’s ‘off’ state, as illustrated in the right inset of Fig. 6b . In both second and third operation, duration of gate pulses determines the amount of protons intercalated in SNO body and further realizes the analogue-state resistivity control. The electrochemical nature of the proton intercalation makes the device’s non-volatile characteristics possible. 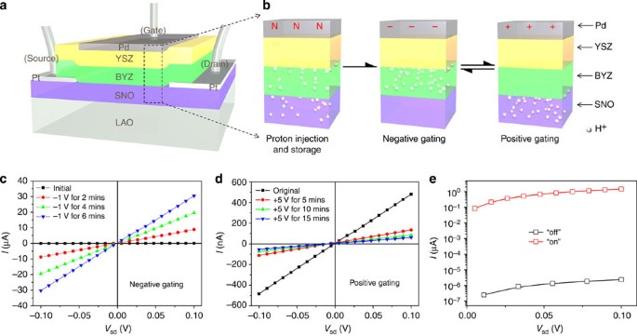Figure 6: Room temperature solid-state proton-gated SNO transistor. (a) Layout of the solid-state proton SNO transistor, where SNO serves as channel layer, BYZ as proton reservoir, YSZ as proton transport barrier at operating temperature and gate insulator, Pd as gate electrode as well as H2dissociation catalyst, Pt as source and drain electrodes. (b) Proposed working principle of the protonic transistor: first, inject protons into BYZ reservoir and SNO channel by H2annealing, illustrated in the left inset ofb; second, extract protons from SNO to BYZ by a negative gating bias, illustrated in the middle inset ofb; third, drive protons from BYZ into SNO by a positive gating bias, illustrated in the right inset ofb. Current versus source–drain voltage of protonic SNO transistor subject to (c) negative gate bias and (d) positive gate bias for different durations. (e) Current versus source–drain bias showing >105on/off ratio. Figure 6: Room temperature solid-state proton-gated SNO transistor. ( a ) Layout of the solid-state proton SNO transistor, where SNO serves as channel layer, BYZ as proton reservoir, YSZ as proton transport barrier at operating temperature and gate insulator, Pd as gate electrode as well as H 2 dissociation catalyst, Pt as source and drain electrodes. ( b ) Proposed working principle of the protonic transistor: first, inject protons into BYZ reservoir and SNO channel by H 2 annealing, illustrated in the left inset of b ; second, extract protons from SNO to BYZ by a negative gating bias, illustrated in the middle inset of b ; third, drive protons from BYZ into SNO by a positive gating bias, illustrated in the right inset of b . Current versus source–drain voltage of protonic SNO transistor subject to ( c ) negative gate bias and ( d ) positive gate bias for different durations. ( e ) Current versus source–drain bias showing >10 5 on/off ratio. Full size image Figure 6c plots the current versus source–drain bias under varied negative gate durations. After 30 s proton injection at 200 °C, the channel resistivity increases from <1 to ~2 × 10 3 mΩ cm. It is found that a large amount of hydrogen gas pockets develop cumulatively during the anodic reaction of SNO under negative gating, which eventually leads to the rupturing of Pd layer [30] . Overloaded protons facilitate this blistering process and underloading helps to prolong the lifetime of the Pd electrode. In real device applications, one may have to tailor the morphology of the electrode to mitigate this effect as is commonly done in the solid-state fuel cell community where noble metal electrodes are routinely used. After initial proton injection, −1 V gate bias with increased duration in geometric sequence (2, 4 and 6 min) is applied. It demonstrates that the channel sheet resistance decreases (from 2.4 × 10 8 Ω per square) drastically in the first 2 min and then slowly afterwards. Eventually, it reduces to 6.6 × 10 5 Ω per square after 6 min gating, which is at least two orders of magnitude in resistivity modulation. Further negative gating is avoided to protect the Pd electrode from blistering by anodic reaction. To demonstrate the ‘turn off’ ability, we operate the device in a narrower modulation window to prevent failure of electrodes. A short negative gate bias pulse is first applied on the as-annealed sample to retract the proton from SNO to BYZ, leading to the sheet resistance value dropping to 4.1 × 10 7 Ω per square. Then a +5 V gate bias with increased duration in geometric sequence (5, 10 and 15 min) was applied ( Fig. 6d ). The resistance in the first 5 min of gating increases quickly at first and increases slowly afterwards, exhibiting a distinct gating rate from the ‘turn on’ process. After 15 min gating, the channel resistance reaches 3.3 × 10 8 Ω per square, demonstrating almost one-order gating capability. By increasing the proton injection time to 15 min and prolonging the negative gating bias to 10 min, five orders of resistivity switching window was realized ( Fig. 6e ). The polarity dependence of channel resistance on gate bias indicates that it is the H + serving as transport carrier. The experimental observations from the operational characteristics of SNO transistor therefore further consolidate our proposed model. The solid-state proton-gated transistor, highlighted by its non-volatility, analogue states and large switching window, room temperature operability could be of further interest for synaptic electronics compatible with CMOS technologies. As these devices can operate over a broad temperature range, they may be monolithically integrated with traditional electronic circuits. We have reported on an electron doping route via chemical methods to realize a phase transition with colossal resistance switching and band gap modulation in a correlated perovskite nickelate. Over eight orders of magnitude on/off ratio in the resistance modulation and an order of magnitude change in optical band gap is demonstrated at room temperature. Independent Li intercalation experiments verifies the proposed model and suggests possible universality of inducing phase transition in nickelates using chemical dopants while preserving parent perovskite crystal structure. We then demonstrate a solid-state proton-gated transistor, which sheds light on the mechanism of resistance modulation and could be of relevance to adaptive and analogue circuits. The ultra-large resistance modulation and the ability to gate the resistance in a solid-state device proximal to room temperature results introduce the nickelates as a semiconductor worthy of consideration for emerging electronic/ionic devices. Synthesis of SNO and Ce-doped SNO Growth of epitaxial and polycrystalline SNO was realized by physical vapour deposition followed by ultrahigh pressure annealing. The ultrahigh pressures are required for thermodynamic phase formation. Before sputtering, the substrate LAO or SiO 2 /Si or Ge wafers was cleaned by acetone, isopropanol and deionized (DI) water and then dried by N 2 gas. For SNO deposition, we utilized co-sputtering with Sm and Ni metal targets. The growth was conducted at 5 mTorr in a constant flow of 40/10 sccm Ar/O 2 mixture with the substrate at room temperature. The d.c. power for the Ni target was adjusted to 75 W and radio frequency power for the Sm target was 150 W to obtain a ~1:1 Sm:Ni cation ratio, as determined by energy-dispersive X-ray spectroscopy. Growth time ranged from 30 min to a few hours to vary the film thickness. The as-sputtered samples were then transferred to a home-built high pressure vessel system. Detailed instrumentation information and thermodynamic conditions for phase formation could be found in ref. 3 . The vessel was then inserted into a tube furnace and ramped to 500 °C for 24 h at 1,500 psi pure O 2 . After annealing, the sample was cleaned by acetone, isopropanol and DI water and then dried by N 2 . A series of Ce-doped SNO samples with different doping concentration were grown on SiO 2 /Si by co-sputtering of CeO 2 , Sm and Ni in Ar/O 2 atmosphere followed by identical high pressure post-annealing procedures as un-doped SNO. Ce concentration was controlled by varying the RF power to the target between 30 and 40 W. Thin film characterization A Zeiss FIB was used to prepare the XTEM sample. Pt (from GIS of FIB) was locally deposited on the TEM lamella to form Pt-SNO-H 2 triple phase boundary. It also serves as a catalyst during H 2 /Ar treatment to enable effective proton intercalation. To anneal the TEM lamella in H 2 /Ar, the TEM grid was horizontally located on a bare SiO 2 /Si substrate and then the whole sample was loaded into the home-built annealing chamber. Across the temperature ramping-up, dwelling and cooling-down processes, the chamber was always fed by the annealing gas. All electron diffraction patterns were acquired when samples completely cooled down to room temperature. XPS characterization was conducted on a K-Alpha Thermo Scientific XPS system, in which the data collection area was fixed to be 200 μm in diameter. The samples were sonicated in acetone, isopropanol and DI water each for 10 min and then blow-dried by N 2 before transfer to the XPS chamber. The angle-dependent, polarization-dependent ellipsometry spectra were obtained using a Woollam WVASE32 instrument at three different angles at wavelengths from 250 to 1,700 nm. The optical constants of LAO substrates were measured from a 1-mm thick bare LAO substrate. The raw ellipsometry data were acquired on the identical SNO on LAO sample before and after hydrogenation. The thickness of the SNO thin film was independently verified by XTEM to avoid over-fitting errors and non-unique solutions. SIMS analysis of pristine SNO, Li-SNO and Mg-SNO samples were conducted at Evans Analytical Group. The experiments were conducted on a Phi Adept 1010 dynamic SIMS tool. The primary ion was O 2+ with the bombardment energy set to be 3 keV. The angle of incidence was 45°. Depth profile was calibrated by TEM combined with SIMS profiling. Lithium-intercalated device fabrication Shadow mask of equally distributed 400 μm diameter holes were used to pattern 100 nm thick Pt electrodes for Ohmic electrical contact and good mechanical adhesion. A drop of saturated lithium perchlorate in propylene carbonate was then dispersed on SNO film. A Li metal plate was anchored above the drop. A positive bias is applied on the metal plate and Pt pad serves as the ground electrode. Solid-state proton transistor fabrication With photolithography, three-terminal SNO transistor devices were fabricated. Dilute hydrogen chloride (3:1H 2 O: HCl) was used to etch SNO. 100 nm thick Pt electrodes were prepared by DC sputtering for Ohmic electrical contact and good mechanical adhesion. BYZ of 60 nm and YSZ of 100 nm were then sputtered on top covering the SNO bar and partial Pt electrodes. Extensive experiments were carried out to determine optimal deposition conditions for the growth of the gate stacks. Both layers were deposited by the magnetron RF sputtering of 100 W with 40 sccm Ar at 5 mTorr. To enable good crystallinity of BYZ, the substrate temperature was adjusted to be 500 °C across BYZ deposition. Substrates were not heated during YSZ deposition. Afterwards, photolithography was used to pattern the Pd gate electrode. E-beam evaporation was used to deposit a thin layer of Pd (40 nm). Electrical measurements Electrical measurements were conducted with a Keithley 2635 A source metre. For resistance–temperature or transistor measurements with SNO device exposed to ambient condition, an environmental probe station (Materials Development Corporation) was utilized. Gate bias was applied with a Keithley 230 voltage supply. To monitor the resistance evolution of SNO during the hydrogenation and O 3 annealing processes, a custom-designed annealing chamber (see Supplementary Fig. 15 ) was used, where H 2 /Ar or O 3 (from an O 3 generator) were regulated to be 150 sccm. This is a crucial piece of equipment setup in a safe fume hood controlled space as performing electrical measurements in ozone at elevated temperatures require great care. Annealing in chlorine gas was conducted at 200 °C for 5 min. Chlorine gas was controlled through a CGA 660 regulator at a flow rate of 100 sccm in a dedicated gas line with new glass container. How to cite this article : Shi, J. et al. Colossal resistance switching and band gap modulation in a perovskite nickelate by electron doping. Nat. Commun. 5:4860 doi: 10.1038/ncomms5860 (2014).